Evolutionary triage governs fitness in driver and passenger mutations and suggests targeting never mutations Genetic and epigenetic changes in cancer cells are typically divided into ‘drivers’ and ‘passengers’. Drug development strategies target driver mutations, but inter- and intratumoral heterogeneity usually results in emergence of resistance. Here we model intratumoral evolution in the context of a fecundity/survivorship trade-off. Simulations demonstrate that the fitness value of any genetic change is not fixed but dependent on evolutionary triage governed by initial cell properties, current selection forces and prior genotypic/phenotypic trajectories. We demonstrate that spatial variations in molecular properties of tumour cells are the result of changes in environmental selection forces such as blood flow. Simulated therapies targeting fitness-increasing (driver) mutations usually decrease the tumour burden but almost inevitably fail due to population heterogeneity. An alternative strategy targets gene mutations that are never observed. Because up or downregulation of these genes unconditionally reduces cellular fitness, they are eliminated by evolutionary triage but can be exploited for targeted therapy. The transition from normal to malignant phenotype during carcinogenesis, often described as ‘somatic evolution,’ is associated with the accumulation of genetic (and epigenetic) mutations [1] , [2] , [3] , [4] but typically demonstrates convergence to common phenotypic properties (the cancer ‘hallmarks’ [5] ). Mutations are commonly characterized as a ‘driver’ or ‘passenger’ depending on the contributions to proliferation and invasion [6] , [7] . Targeted therapies can produce significant tumour response by disrupting driver mutations. However, not all tumours have identifiable and/or drugable driver mutations and response to targeted therapy, even when the driver mutation is present, is usually transient as resistant phenotypes repopulate the tumour [8] . Here we investigate genetic heterogeneity, phenotypic convergence, the conventional binary classification of driver/passenger mutations and corresponding targeted therapy in the context of Darwinian dynamics. This extends ongoing efforts to understand cancer from first principles on the basis of evolution by natural selection [9] , [10] , [11] , including the classical trade-offs observed in Darwinian systems. Here, we consider a multi-loci diallelic model of mutation and selection within a finite population of tumour cells evolving along a well-defined adaptive landscape. In examining the evolutionary dynamics during carcinogenesis, we assume that normal epithelial cells exist in an evolutionary and ecological state well below their maximal carrying capacity and individual evolutionary potential for survival and proliferation. That is, normal cells carry out their differentiated tasks for maintaining whole organism function and their population density, survival and proliferation is entirely controlled by tissue signals. Ecologically, a new cancer cell lineage begins with abundant available space (the lumen of a duct, for example) and is initially free from the life history trade-off of proliferation versus survivorship. Evolutionarily, the tumour lineage develops a self-defined fitness function, and then uses the human genome to evolve strategies to enhance survival and/or proliferation. Consistent with the fundamental laws of evolution, each population may initially undergo exponential proliferation but is ultimately ecologically constrained by the limitations of substrate and space. Here, the evolutionary trajectory reaches the classical Darwinian life history trade-off [12] , [13] , in which cancer cells must invest limited available resources in some combination of survival and fecundity that maximizes fitness within the context of their environment. These phenotypic strategies are apparent in the consistent convergence to the ‘hallmarks’ of cancer. We use in silico simulations based on Darwinian first principles and classical evolutionary trade-offs to investigate the genomic dynamics that are both a cause and consequence of tumour development and progression. Our specific interests focus on the conventional designation of driver and passenger mutations, the source of observed spatial intratumoral heterogeneity, and the dynamics of tumour response and resistance to targeted therapies. Our results demonstrate that the fitness value of most genetic and epigenetic events are contextual and depend on extant environmental selection forces, other local populations and the prior evolutionary arc of the cell—dynamics that we collectively describe as ‘evolutionary triage.’ We find that, as a result of evolutionary triage, the same mutation can act as passenger or driver depending on context. In a stable microenvironment, evolutionary triage will reduce tumour cell diversity so that the observed intratumoral molecular heterogeneity is largely due to the variations in local selection pressures caused by, for example, blood flow. Our results demonstrate a previously unrecognized therapeutic target—‘never’ mutations. That is, when a gene is never or rarely observed to be mutated, we must conclude that up or downregulation of that gene unconditionally reduces cell fitness. We demonstrate that targeting never genes can be a highly effective therapeutic strategy. Evolutionary triage Pooling genetic data from the 225 carcinogenesis simulations, we observed 3,334 unique genotypes (5.09% of all possible genotypes) within the evolving cancers. Although the model randomly imposed mutations on each gene, the frequency with which each mutation was observable in the tumour was strongly influenced by its associated fitness change—a phenomenon we term ‘evolutionary triage.’ The observed frequency of neutral mutations is 0.6% per generation and at least one neutral mutation is found in ~25% of the cells in the final tumour populations. Thus, the observed frequency of passenger mutations per generation permits, as expected, a reasonable estimate of the actual mutation rate (which was 1% in our simulations). In some simulations, a neutral allele ‘hitchhiked’ with a successful mutation and formed temporary linkage disequilibrium ( Figs 1 and 2 ) so that it was present in a frequency greater than expected. 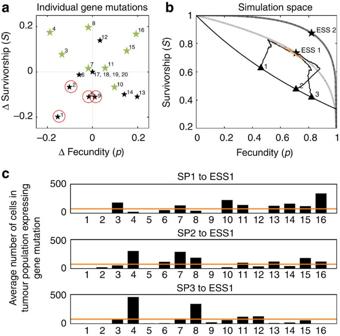Figure 1: Evolutionary trajectories and gene prevalence. (a) During evolution to ESS1 (Evolutionary Stable State 1), the genes highlighted in green conferred increased fitness depending on the starting initial phenotype. The genes circled in red, such as gene 1, reduce both fecundity and survivorship and were never observed in the final simulated cancer populations. (b) Multiple evolutionary trajectories exist to ESS1 depending on the initial phenotype. This functional equivalence results in genetic heterogeneity within and between patients as seen inc. (c) The mutation prevalence varies greatly depending on the initial phenotype. The orange line represents the neutral mutation prevalence. Figure 1: Evolutionary trajectories and gene prevalence. ( a ) During evolution to ESS1 (Evolutionary Stable State 1), the genes highlighted in green conferred increased fitness depending on the starting initial phenotype. The genes circled in red, such as gene 1, reduce both fecundity and survivorship and were never observed in the final simulated cancer populations. ( b ) Multiple evolutionary trajectories exist to ESS1 depending on the initial phenotype. This functional equivalence results in genetic heterogeneity within and between patients as seen in c . ( c ) The mutation prevalence varies greatly depending on the initial phenotype. The orange line represents the neutral mutation prevalence. 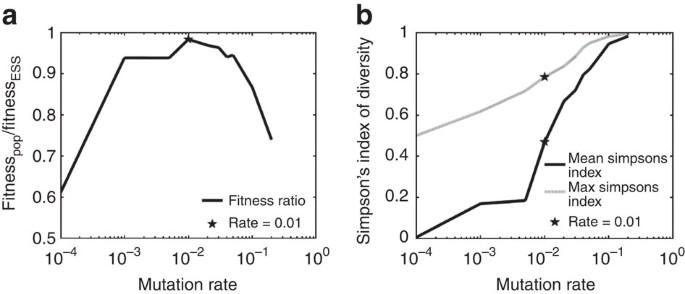Figure 2: Effect of different mutation rates. (a) Theyaxis shows the ratio between the mean fitness reached by the population after 2,000 generations and the fitness achievable at the ESS (SeeFig. 2b). For this example, we used ESS 1 with a maximum fitness=0.3). Thexaxis varies the mutation rate with units of mutation/cell/division with the lowest value slightly higher than that of normal cells35. With a low mutation rate, the evolution is too slow to reach the ESS. As the mutation rate increases (between 10−3and 10−1), the tumour population evolves to the ESS. However, at very high mutation rates, the population is unstable and fitness decreases due to a mutation/selection balance—a phenomenon predicted by Haldane34. (b) Here, we demonstrate that the diversity (but not necessarily fitness as shown in panela) of tumour populations increases with mutation rate. For the remaining simulations, we chose a mutation rate of 10−2(star) as the midpoint between these trade-offs. Full size image Figure 2: Effect of different mutation rates. ( a ) The y axis shows the ratio between the mean fitness reached by the population after 2,000 generations and the fitness achievable at the ESS (See Fig. 2b ). For this example, we used ESS 1 with a maximum fitness=0.3). The x axis varies the mutation rate with units of mutation/cell/division with the lowest value slightly higher than that of normal cells [35] . With a low mutation rate, the evolution is too slow to reach the ESS. As the mutation rate increases (between 10 −3 and 10 −1 ), the tumour population evolves to the ESS. However, at very high mutation rates, the population is unstable and fitness decreases due to a mutation/selection balance—a phenomenon predicted by Haldane [34] . ( b ) Here, we demonstrate that the diversity (but not necessarily fitness as shown in panel a ) of tumour populations increases with mutation rate. For the remaining simulations, we chose a mutation rate of 10 −2 (star) as the midpoint between these trade-offs. Full size image In Fig. 1 , we demonstrate that the fitness advantage gained by mutations (green) conferring an increase in fecundity and/or survival allowed the cells with these mutations to proliferate more frequently. Consistent with the clinical observations, driver genes are observed with far higher frequency (up to 92%) in the final tumour populations although with considerable variability. Finally, mutations in genes (red) that resulted in a decrease of survival and or fecundity were observed during all of our simulations but became extinct quickly due to the fitness disadvantage. Their frequency in the final tumour was invariably near or equal to 0. The basal cancer mutation rate This study primarily examines the effects of evolutionary triage variations on the observed mutation rate in each gene. However, in identifying a basal mutation rate ( Fig. 2 ), we gained the unexpected insight that cancer evolution requires a ‘goldilocks’ mutation rate. Specifically, a mutation rate that is too low (<10 −3 ) will not allow adequate exploration of the adaptive landscape and will result in a small, homogeneous and effectively ‘benign’ tumour. On the other hand, a mutation rate that is too high (>0.1) produces a mutation-selection balance in which fitness-reducing mutations occur too rapidly to be eliminated resulting in an overall decline in fitness and failure to reach the ESS. These dynamics could potentially be exploited for cancer prevention or treatment although this is beyond the current scope of the manuscript. Intratumoral molecular heterogeneity In Fig. 3 , we quantified tumour heterogeneity over time using the Simpson’s Index of Diversity (SID) which gives the probability that two randomly chosen tumour cells have different genotypes. A value close to 0 indicates very little genetic variability and a value of 1 indicates that all individuals have a unique genotype. 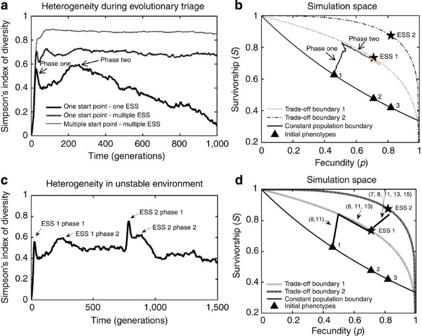Figure 3: Simpson’s Index of Diversity. We demonstrate that heterogeneity of intratumoral phenotypes will vary as tumour populations evolve along the adaptive landscape. (a) The Simpson’s Index of Diversity is shown for stable or spatially varying landscapes. The solid line marked corresponds to the trajectory (b), in which there is a single, stable ESS. Initial somatic evolution results in a rapid increase in heterogeneity as the early tumour moves toward the trade-off boundary. However, during later evolution, the intratumoral populations decrease in heterogeneity as the tumour moves closer and closer to the maximal fitness point, ESS1. This predicts that tumour cells in a stable environment will exhibit on limited diversity. In contrast, for spatially complicated landscapes (c,d), for example, due to temporal and spatial variations in blood flow, heterogeneity remains high (c). The results suggest that the observed heterogeneity in tumour largely reflects variations in environmental selection forces (that is, vascular density and blood flow). Similar temporal variations during tumour development were predicted in (ref.2). Figure 3: Simpson’s Index of Diversity. We demonstrate that heterogeneity of intratumoral phenotypes will vary as tumour populations evolve along the adaptive landscape. ( a ) The Simpson’s Index of Diversity is shown for stable or spatially varying landscapes. The solid line marked corresponds to the trajectory ( b ), in which there is a single, stable ESS. Initial somatic evolution results in a rapid increase in heterogeneity as the early tumour moves toward the trade-off boundary. However, during later evolution, the intratumoral populations decrease in heterogeneity as the tumour moves closer and closer to the maximal fitness point, ESS1. This predicts that tumour cells in a stable environment will exhibit on limited diversity. In contrast, for spatially complicated landscapes ( c , d ), for example, due to temporal and spatial variations in blood flow, heterogeneity remains high ( c ). The results suggest that the observed heterogeneity in tumour largely reflects variations in environmental selection forces (that is, vascular density and blood flow). Similar temporal variations during tumour development were predicted in (ref. 2 ). Full size image We used the SID as virtual data in an analysis of variance between groups (ANOVA) with starting point (three initial conditions), end point (ESS1, ESS2, ESS2 via ESS1, and intratumoral areas of ESS1 and ESS2), and generation (35, 60, 100 and 1,000) as independent variables. The analyses were performed in Systat [12] (see Supplementary Table 1 ). Our virtual patients were nested within the starting point by end-point combinations, and we examined the three two-way interactions between independent variables. All main effects and interaction effects were significant. This statistical model demonstrates that ~60% ( r 2 =0.588) of the variation between patients can reflect variations in the properties of the adaptive landscape. However, patients frequently differed significantly from each other independent of the starting conditions or ending ESS (F 288,882 =1.65, P <0.001), suggesting that early mutations and evolutionary trajectories remained persistent within a given patient over time. Figure 3a demonstrates that increased genetic variability occurs consistently early in carcinogenesis because the initial population grows with little inter- or intraspecific competition (F 3,882 =19.10, P <0.001). That is, as the early populations expand into unoccupied space (the lumen of a duct or colon, for example) any genotype conferring higher fitness than the original normal population will proliferate. This first phase ends when the proliferation becomes limited by space and substrate and the tumour population evolves along the fecundity–survival trade-off boundary. As shown in Fig. 3 , these Darwinian forces selects for the relatively small number of genotypes that confer maximal fitness and the population becomes more homogeneous as a small number of genotype-specific populations dominate. Furthermore, there is strong selection against any new genotype because no available strategy is fitter than the extant population. Thus, when tumour populations reach a fitness maximum, the observed mutation rate becomes effectively 0. In contrast, tumours with spatially varying landscapes (in which, for example, ESS1 and ESS2 ( Fig. 3a ) exist within the same tumour) or temporally varying landscapes (in which the entire tumour transitions from ESS1 to ESS2 ( Fig 3c,d )) maintain increased molecular heterogeneity when compared with a single, stable ESS environment (F 3,288 =105.6, P <0.001). These results suggest that the observed molecular heterogeneity within tumours, rather than an unpredictable manifestation of random mutations, is dependent on variations in environmental selection forces, such as blood flow, and could be observed and predicted by clinical imaging [13] . Evolutionary triage governs driver and passenger mutations Driver mutations are defined as those that confer a proliferative advantage and are causally implicated in carcinogenesis [14] . However, the simulation results demonstrate that identifying true driver mutations from an observed data set is difficult. 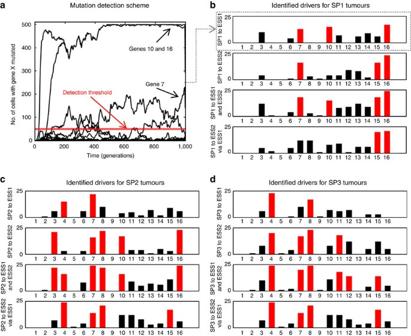Figure 4: Identifying driver mutations. (a) The gene mutation prevalence for one patient (initial phenotype 1 to ESS1) is shown. The ‘biopsy’ occurs at the end of simulation, at 1,000 generations. We assume that if at least 10% of the cells in the whole tumour exhibit a mutation in a particular gene at the time of biopsy, it will be detected. In this particular biopsy, mutations in genes 7, 10 and 16 would be identified. (b–d) This biopsy detection scheme is conducted for all patient samples and each detection is tallied. If a mutation in a particular gene is detected in at least 12 of the patients, it is highlighted in red. Figure 4 shows data from ‘virtual biopsies’ of 25 patient tumours for 12 possible evolutionary trajectories from normal to cancer. Although a mutation in every gene is detectable in at least one patient ‘biopsy’, with the exception of gene 1, many of the mutations only occur in a minority of the cohort so that only two to four potential drivers are observed in ≥50% of the simulated patients within each group. These findings are consistent with the observations of ‘hotspots’ in the cancer genome in which there is apparently an increased mutation rate [15] . Figure 4: Identifying driver mutations. ( a ) The gene mutation prevalence for one patient (initial phenotype 1 to ESS1) is shown. The ‘biopsy’ occurs at the end of simulation, at 1,000 generations. We assume that if at least 10% of the cells in the whole tumour exhibit a mutation in a particular gene at the time of biopsy, it will be detected. In this particular biopsy, mutations in genes 7, 10 and 16 would be identified. ( b – d ) This biopsy detection scheme is conducted for all patient samples and each detection is tallied. If a mutation in a particular gene is detected in at least 12 of the patients, it is highlighted in red. Full size image Thus, in each case, frequently observed mutations represent drivers that increase fitness and are causal in the transition of that cell from normal to cancer. However, in every cohort and in every tumour, some tumour cells achieved a maximally fit phenotype through less common combinations that reflect different genetic trajectories generated by chance or by environmental variations. For example, the mutation combination as observed in refs 8 , 11 confer virtually the same overall change in fecundity and survivorship as the mutation combination observed in refs 10 , 16 . In tumours from initial phenotype 1 to ESS1, mutations 8 and 11 might be incorrectly viewed as of limited importance because they are relatively infrequently expressed. These results are consistent with previously recognized limitations in the identification of driver mutations from clinical data sets. However, our model results also demonstrate that conventional definitions of driver mutations should include an evolutionary and ecological context. Specifically, we find that the fitness value of any mutation qualitatively and quantitatively varies depending on: 1 The initial normal phenotype; mutations in gene 4, which is a ‘driver’ for cells originating from initial phenotype 3, are deleterious or ‘passenger mutations’ for cells originating from phenotype 1. 2 The local environment both present and past; evolution from phenotype 2 towards ESS1 selects for mutations in genes 4 and 7, while evolution from the same initial phenotype towards ESS2 selects for 3, 7, 8, 10 and 16. Gene 16 is strongly selected when initial phenotype 2 evolves to ESS2 but is rarely seen in tumours that first evolved to ESS1 and then transitioned to ESS2. 3 Prior mutational history. From initial phenotype 1 to ESS2, mutations in genes 15 and 16 confer the greatest fitness advantage. However, if a mutation in gene 8 first occurs, genes 15 and 16 become deleterious mutations and are not observed ( Supplementary Fig. 1 ). Evolutionary triage and targeted therapy Figures 5 and 6 present simulation results from targeted therapy. In Fig. 5 , therapy targets gene 16 which is the most commonly mutated gene in all evolutionary trajectories ( Fig. 4 ). For example, in simulations of 75 patient tumours evolved from each start point to ESS1, a complete and prolonged reduction in tumour burden was achieved in 9%. In 56.0% patients, targeted therapy achieves a significant response followed by adaptation and proliferation of resistant populations. In 28.0%, no reduction in tumour volume is observed although size stabilization with some delay in progression was observed in 7%. Resistance in our model occurs when cancer cell lineages that evolved without the target gene (often sparsely represented in the initial population) gain an adaptive advantage due to suppression of the dominant population and proliferate rapidly. Because of supervenience [16] , alternative gene combinations replace and then evolve to maximize fitness. 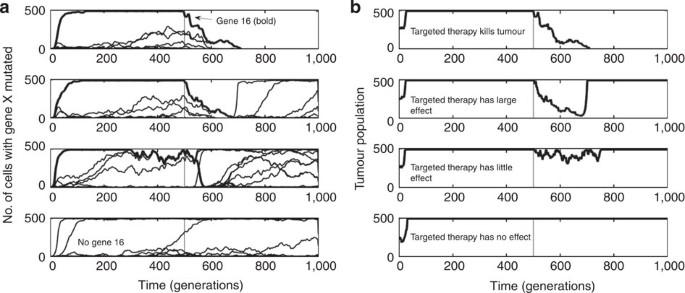Figure 5: Mutation prevalence and population dynamics of tumours from initial phenotype 1 during targeted therapy simulation. (a,b) The underlying mutational prevalence for four representative tumours are shown inawhile the corresponding population dynamics are shown inb. At the time of treatment (generation 500), the prevalence of mutation 16 drops to zero. After treatment, if the tumour survives, the evolutionary strategies used to reach maximal fitness can be observed. The top example shows the dynamics in 9.3% patients where a full response to therapy is observed. The second shows a representative moderate response with eventual proliferation of resistant populations. The third shows a delay in progression though no significant response. The last example shows how in 28% patients, the therapy had no effect. Figure 5: Mutation prevalence and population dynamics of tumours from initial phenotype 1 during targeted therapy simulation. ( a , b ) The underlying mutational prevalence for four representative tumours are shown in a while the corresponding population dynamics are shown in b . At the time of treatment (generation 500), the prevalence of mutation 16 drops to zero. After treatment, if the tumour survives, the evolutionary strategies used to reach maximal fitness can be observed. The top example shows the dynamics in 9.3% patients where a full response to therapy is observed. The second shows a representative moderate response with eventual proliferation of resistant populations. The third shows a delay in progression though no significant response. The last example shows how in 28% patients, the therapy had no effect. 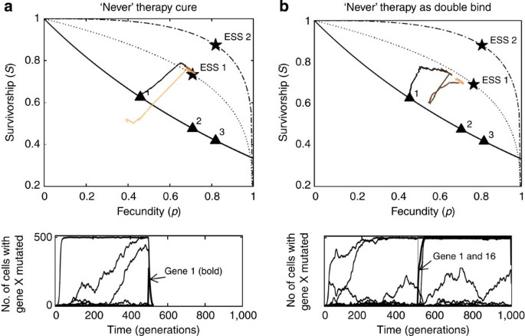Figure 6: ‘Never’ therapy outcomes. (a) On the left, the evolutionary trajectory to ESS1 from the initial phenotype 1 is shown in black. After the ‘never’ therapy is administered, the trajectory falls below the sustainability line and results in tumour extinction, shown in orange. More commonly, the ‘never’ therapy does not cause tumour eradication but because cells with mutated gene 16 survive and remain sufficiently fit to proliferate and repopulate the tumour (b). This represents a classical treatment ‘double bind’30and renders the tumour exceedingly susceptible to the traditional targeted therapy directed against driver gene 16. In 80% simulations, this strategy produced complete tumour eradication. Full size image Figure 6: ‘Never’ therapy outcomes. ( a ) On the left, the evolutionary trajectory to ESS1 from the initial phenotype 1 is shown in black. After the ‘never’ therapy is administered, the trajectory falls below the sustainability line and results in tumour extinction, shown in orange. More commonly, the ‘never’ therapy does not cause tumour eradication but because cells with mutated gene 16 survive and remain sufficiently fit to proliferate and repopulate the tumour ( b ). This represents a classical treatment ‘double bind’ [30] and renders the tumour exceedingly susceptible to the traditional targeted therapy directed against driver gene 16. In 80% simulations, this strategy produced complete tumour eradication. Full size image These results for targeted therapy are consistent with clinical observations and conventional explanations for the results [17] , [18] . Does evolutionary triage suggest an alternative treatment strategy? Recall that, as a result of evolutionary triage, mutations that confer a decrease in fitness are virtually never observed in advanced cancers. We hypothesized that these genes might represent potential therapeutic targets. In our simulation, gene 1 confers a negative change in both survivorship and proliferation. As a result, gene 1 would never be considered a potential therapeutic target. Figure 6 shows the effect of a therapy that effectively upregulates gene 1 in a tumour population originating from initial phenotype 1 to ESS1. We see that the forced upregulation of this gene can push tumour population fitness <0 from ESS1 and results in complete extinction of the tumour population. The success of therapy demonstrates that, for ‘never gene’ targets, every tumour cell is susceptible. Thus, although the simulations do not demonstrate complete extinction in every case (because some of the diverse tumour genotypes can overcome the negative fitness effects), all tumours were significantly affected. Interestingly, combinations of therapy targeting driver and ‘never’ mutations were consistently successful in causing complete tumour eradication because adaptations to the ‘never’ therapy required marked upregulation of one driver gene, in particular, gene 16 ( Fig. 6b ). When applying solely the targeted therapy, only 9% of tumours were completely eradicated. Remarkably, when all tumours are first given the ‘never gene’ upregulation therapy followed by the targeted therapy on gene 16, 80% of the tumours were completely eradicated. This is an example of an evolutionary double bind therapy, where an initial therapy forces a precise evolutionary reaction, in this case an upregulation of gene 16, which is specifically treatable by the secondary therapy [19] . Our goal in this work is to contribute to the development of a Darwinian theoretical framework for the large and often confusing molecular data sets generated by cancer biologists and oncologists. Recently, Weinberg, writing in a Cell commentary [20] , observed that the common genetic paradigm of cancer ‘has reigned supreme for four decades’ but he advocated a ‘move back to confronting the endless complexity of the disease.’ He concluded: ‘… it is becoming increasingly apparent that a precise and truly useful understanding of the behavior of individual cancer cells and the tumors that they form will only come once we are able to integrate and then distill these data’. In a 2013 Nature article [21] , we wrote, ‘Ultimately, real progress in understanding cancer biology will require a formal intellectual framework. Like gravity or quantum field theory in the physical sciences, we must define the underlying principles governing the nonlinear dynamics that give rise to the vast and complex data sets being generated by the creative minds of molecular biologists. These principles will not be found until we begin to search in the right place.’ Here we examine Darwinian dynamics as the unifying first principles of cancer and use a classical evolutionary trade-off to clarify the molecular heterogeneity found in most cancers. The proposed evolutionary dynamics are not explicitly genetic. We focus on phenotypic interactions with environmental selection forces and view genetics as the ‘mechanism of inheritance.’ However we show that this approach is entirely compatible with the molecular data and provides both organizing principles and novel insights. Our results demonstrate that the extensive genetic data sets now available in cancer need to be understood in the context of ‘evolutionary triage’ which governs the frequency with which any molecular property is observed. That is, following a random genetic or epigenetic change in a cancer cell, proliferation of the resulting phenotype is dependent on the fitness effect which is, in turn, governed by the prior genetic trajectory of the cell, local environmental selection forces, and the extant populations. Thus, the distribution of observed mutations can be used to understand and simulate evolutionary and ecological dynamics within a tumour. Here, we use models based on the evolutionary triage principle to examine current concepts of driver and passenger mutations, the source of intratumoral molecular heterogeneity and the efficacy of targeted therapy. Our simulations produce molecular heterogeneity within tumour populations that is similar to clinical observations. Our simulations demonstrate that this diversity is not an inevitable result of accumulating mutations but rather a consequence of variable selection forces due to environmental heterogeneity caused, for example, by variations in blood flow. In fact, our simulations find that, due to evolutionary triage, the diversity of tumour populations and the apparent mutation rate within a stable region will significantly decline after reaching a fitness maximum. Our model also demonstrates that mutations that confer an increase in fitness will be observed with higher frequency than those that do not, consistent with the general bimodal classification of drivers and passengers. However, we find that accurate designation of driver or passenger mutation is possible only when the evolutionary and ecological context is known. That is, some mutations may be drivers in one environment but not in another. This context dependence has been experimentally observed in the Wilms' tumour 1 (WT1) gene [18] . Furthermore, the state of the cell along the genetic trajectory is critical so that a mutation can be a driver early in the evolutionary process but may not confer an equal adaptive advantage in later stage cells. In general, this demonstrates the principle of supervenience or functional equivalence [10] , [22] in which cancer cells exhibit phenotypic convergence (that is, the hallmarks) but through multiple different genetic trajectories resulting in genotype divergence. Finally, our results demonstrate that therapy targeted to commonly observed mutations (regardless of their designation as driver or passenger) will generally reduce the population and occasionally produce a complete and prolonged response. However, uncommon extant populations that achieve maximal fitness through some other genetic trajectory are virtually always present and eventually permit tumour progression. This is consistent with the results of targeted therapies in lung cancer and melanoma [23] , [24] . Perhaps the most non-intuitive prediction of the evolutionary triage model is that mutations that are never or rarely observed may provide a more consistent and durable response. This builds on prior results that used information theory to demonstrate that changes in critical genes cannot be observed in a Darwinian environment [25] . These mutations are, thus, eliminated by evolutionary triage because their normal function is necessary to maintain cancer cell fitness and thus both up and downregulation unconditionally results in a decrease in fitness. Interestingly, systematic investigation of knockout mutants in Escherichia coli found that ~10% of genes were indispensable but this could vary considerably based on the culture conditions [26] , [27] . This dependence on microenvironmental conditions is consistent with our general results that the fitness value of a gene (whether driver, passenger or never) will depend on the critical selection forces within the environment, which can vary. To further investigate this, we searched the Cancer Genome Atlas (TCGA) data sets for genes that are not listed. This demonstrated that 1,100 genes of 20,000 protein coding genes (5.5%) are not mutated in any of the TCGA data sets (total of ~4,400 patients). The prediction that targeting never genes can be an effective therapy will require explicit investigation to confirm or refute. We do note, however, that while the proximal components of the MAPK pathway (EGFR, RAS and RAF) are ‘driver’ mutations, gain or loss of function mutations in the distal components, MEK and ERK, are rarely observed. The obvious strategy is blocking a never gene and both MEK and ERK inhibitors are under investigation [28] , [29] . However, a less obvious strategy is upregulating MEK expression. While this initially seems counter-intuitive, the simple observation that such a mutation is not observed in cancer suggests that overexpression of MEK also reduces fitness in a tumour environment (probably because unmodified proliferative signals will produce mitosis in inadequate environmental conditions leading to cell death). Our results suggest a counter-intuitive approach in which therapy that increase activity of MEK, ERK and other distal components of pathways may be a highly effective therapy. Finally, our model also suggests that combination therapies sequentially targeting a never mutation followed by targeting a compensating driver mutation may be substantially more effective than either treatment alone. Finally, we note that sequential therapy targeting first a never mutation followed by treatment of a classic driver phenotype had a high probability of eliminating the entire cancer population. This is because the tumour cells that were adapted to the first therapy universally required the driver mutation to maintain fitness—a therapeutic strategy classified as ‘double bind [30] ’. Fecundity and survivorship trade-off We model carcinogenesis within the classic evolutionary life history trade-off: fecundity versus survivorship [31] , [32] , [33] , [34] . This trade-off becomes inevitable in any evolving population. As tumour cell populations grow and compete, cells can either increase life span through survival strategies that promote longevity at the cost of a reduced reproduction rate, or vice-versa. But, simultaneous increase in both is impossible [31] , [32] , [33] . A cell’s fitness (per capita growth rate) is given as: where S is the probability of surviving, and p is the probability of undergoing cell division. The term in brackets represent the finite growth rate of a cell on the basis of its probability of dying and/or dividing in a given time step (often denoted as λ in models of population growth [35] ), and the logarithm of the finite growth rate gives the instantaneous per cell growth rate, where x is the population size of tumour cells. The formulation of this fitness function is described in Fig. 7c . Note S and p combine several cancer ‘hallmarks’ [5] as p is governed by self-sufficiency from growth signals and insensitivity to anti-growth signals and S represents evasion from apoptosis and replicative immortality. 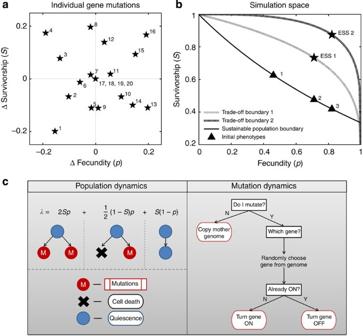Figure 7: Simulation setup. (a) Each of the 16 mutations confers a unique change to fecundity and survivorship. For example, mutation 16 increases both fecundity and survivorship a large and equal amount while mutation 9 greatly decreases survivorship but has no effect on fecundity. Mutations 17–20 true passenger mutations, conferring no change in survivorship or fecundity. (b) Normal cells are found on the solid line, with the three specific normal populations used in the simulations highlighted (triangles). When carcinogenesis is allowed, cells evolve from their original phenotype toward the dotted lines which represents the trade-off between survivorship and fecundity above which cells require too many resources, and are unable to survive. The point at which the fitness of an evolving cell within the extant environment is maximized is highlighted (stars). The path from a starting point to the maximization point corresponds to somatic evolution during carcinogenesis and represents acquisition of the hallmarks of cancer outlined in the text. (c) Our fitness formulation assumes three distinct cell outcomes for each generation. (1) A cell can divide, allowing mutations in both mother and daughter, (2) a cell can survive first and then may divide (death precedes cell division) or divide first and then the progenitor cell may die (cell division precedes death) and (3) a cell may continue to the next generation. The mutation dynamics outline the process by which a mutation event is determined. Figure 7: Simulation setup. ( a ) Each of the 16 mutations confers a unique change to fecundity and survivorship. For example, mutation 16 increases both fecundity and survivorship a large and equal amount while mutation 9 greatly decreases survivorship but has no effect on fecundity. Mutations 17–20 true passenger mutations, conferring no change in survivorship or fecundity. ( b ) Normal cells are found on the solid line, with the three specific normal populations used in the simulations highlighted (triangles). When carcinogenesis is allowed, cells evolve from their original phenotype toward the dotted lines which represents the trade-off between survivorship and fecundity above which cells require too many resources, and are unable to survive. The point at which the fitness of an evolving cell within the extant environment is maximized is highlighted (stars). The path from a starting point to the maximization point corresponds to somatic evolution during carcinogenesis and represents acquisition of the hallmarks of cancer outlined in the text. ( c ) Our fitness formulation assumes three distinct cell outcomes for each generation. (1) A cell can divide, allowing mutations in both mother and daughter, (2) a cell can survive first and then may divide (death precedes cell division) or divide first and then the progenitor cell may die (cell division precedes death) and (3) a cell may continue to the next generation. The mutation dynamics outline the process by which a mutation event is determined. Full size image Pre-malignant initial conditions We chose three different starting values for S and p ( Fig. 7b ). They simulate the effects of genetic and epigenetic variability in normal and pre-malignant cells due to random mutations, environmental factors, such as chronic inflammation, or germ line variations in different individuals. The initial values of S and p for these three initial conditions were set to just allow cells to replace individuals that are lost. This maintains a regulated, stable and sustainable population of normal cells. Genetic mutations Normal cells evolve toward a malignant phenotype by stochastically accumulating mutations at any of the 16 gene loci. We treat all gene mutations as haplotypes and permit just two haplotypes per locus: wild-type (state of normal cell) or mutated (not present in the normal cells). In the simulations, 22 genes were examined. Of these, four did not affect either fecundity or survivorship and served as neutral or passenger genes. Sixteen ‘active’ (i.e. altered the cell fitness) genes each conferred a unique change in survival, S, and fecundity, p ( Fig. 7a ), resulting in (2 16 ) 65,536 possible combinations of cumulative changes in S and p ( Supplementary Fig. 2 ), and two genes resulting in immediate cell death. The computer code used in the study and the raw data from simulations are available at https://github.com/cunninghamjj/Evolutionary-triage-in-Cancer . The location of the 16 genes in the fecundity and survivorship landscape were created using a randomizing algorithm under two rules; (1) four genes must lie in each quadrant and (2) the range for both fecundity and survivorship will fall between −0.2 and 0.2, which is the mean distance between the values of normal cells and the tumour ESS sites. As shown in Supplementary Figs 2 and 3 , with these methods, 16 active genes were the minimum number sufficient to allow genetic access to cover the relevant evolutionary adaptive landscape. Fewer than 16 resulted in patchy inconsistent coverage and more than 16 showed diminishing returns of landscape coverage versus computational requirement ( Supplementary Fig. 3 ). In multiple simulations, we find that the locations of these 16 genes will affect the specifics of the results, such as which genes are ‘drivers’ and which combine to create successful combinations. However, it does not affect the overall conclusions pertaining to heterogeneity. In our simulations, four genes moved the cellular fitness toward higher values of both S and p and four other genes increase either just fecundity or just survivorship. These represent potential ‘drivers’ in that they can increase fitness within the adaptive landscape. More genes could be added at the price of increased complexity and computational time. However, the simulation seemed consistent with recent analysis of genomic changes in different cancer types [36] , [37] that found two to eight driver mutations in most tumours. The other genes either have no effect (that is, classic passengers) or a negative effect on fitness. Evolutionary stable strategies In our model, two maximal fitness [ S, p ] points on the [ S, p ] trade-off boundaries ( Fig. 1b ) represent different adaptive landscapes due to, for example, regional variations of blood flow. The boundary is defined by the following equation: We view one fitness maximum as a well-vascularized, nutrient-rich area selecting for greater investment in proliferation ( α =1, β =4) resulting in ω ( S , p )=0.2996, whereas the second fitness maximum is an area of diminished blood flow selecting for greater investment in survival ( α =3, β =6) resulting in ω ( S , p )=0.3005. Evolution from one of the three initial conditions to one of the two maximal fitness points requires different evolutionary trajectories reflecting variations in selection pressures. These fitness maxima were not selected arbitrarily but represent the evolutionarily stable strategies (ESS of Maynard Smith [38] ) that emerge from letting the tumour cells engage in an evolutionary game in which each cell’s fitness-maximizing strategy depends upon the strategies of the other cells [39] . Two limits are imposed upon the evolving tumours: a carrying capacity and the fecundity versus survivorship trade-off. The former represents proliferation limitations due to restrictions in space and substrate and is simulated by randomly culling cells when the population exceeds its carrying capacity. The latter is imposed by the fitness landscape ( Fig. 7 ). Mutation rate Although simple, we favour this model for three reasons. First, it follows the pattern of reproduction used by cancer cells, which, as clonal propagators, lack meiosis and the Mendelian properties of segregation and independent assortment. Second, the altered genetics are not only a product of explicit mutations, but could also result from regulator genes, heritable epigenetic changes, other coding genes and/or gene duplications and deletions. Third, while simplifying to two gene states at 16 loci offers many fewer ‘degrees of freedom’ than the genome of a cancer cell, it is consistent with the number of driver genes typically observed in a wide range of cancers, and it allows us to follow explicit gene states. We recognize that reversal of each actual mutation is ordinarily viewed as improbable, but has been well documented in a wide range of organism traits [40] . Furthermore, the reversal of the phenotypic consequence of most genetic changes can occur when the environmental selection forces change. A simple example is the reversal of the MDR phenotype in vitro when chemotherapy is removed from the culture media [22] . In the simulations presented here, we used a mutation probability of 0.01 per cell per division. When a mutation event occurred, it was randomly assigned to one of the 16 genes. The actual mutation rate in cancer cells is not well established and hence a controversial topic. The estimated or measured number of mutations per cell per division varies widely. In fact, one motivation for this work was to examine variations between the actual underlying mutation rate and the observed mutation rate in each gene as a result of evolutionary triage. In our preliminary work ( Fig. 2 ), we found that the results were unaffected by using mutation rates that were an order of magnitude lower or higher than 0.01. With a mutation rate >10%, the cell lineages cannot stay at the ESS due to wandering from a mutation-selection balance [23] , whereas substantially lower mutation rates (10 −4 ) made evolution too slow for achieving the ESS even after 2,000 generations. The value is greater than that typically observed in normal cells [24] and in the general range of estimated cancer mutation rates observed in other studies [41] . Thus, the choice seemed biologically reasonable and, importantly, allowed computational efficiency without loss of general applicability. Simulations and replications We simulated cancer development during 1,000 cell generations (representing 3–10 years depending on the rates of cell division) in ‘patients’ under the nine simulation permutations with 25 replicates for a total of 225 ‘patients’. The nine reflect the three starting phenotypes and three possible evolutionary trajectories (ESS1, ESS2 and transition from ESS1 to ESS2 due to temporal variations in blood flow; Supplementary Fig. 1 ). Once tumours are established, we simulated targeted therapy by assuming that the resulting change in a driver gene renders the cell non-replicative and imposes a specific mortality rate of 25% per generation time. In addition, the dynamics of therapies targeted to ‘non-driver’ genes and combinations of therapies can be analysed. Nine hundred simulated patients were analysed for this model (data available at http://tinyurl.com/ntslsy8 ). How to cite this article: Gatenby, R. A. et al . Evolutionary triage governs fitness in driver and passenger mutations and suggests targeting never mutations. Nat. Commun. 5:5499 doi: 10.1038/ncomms6499 (2014).